PI3K–GSK3 signalling regulates mammalian axon regeneration by inducing the expression of Smad1 In contrast to neurons in the central nervous system, mature neurons in the mammalian peripheral nervous system (PNS) can regenerate axons after injury, in part, by enhancing intrinsic growth competence. However, the signalling pathways that enhance the growth potential and induce spontaneous axon regeneration remain poorly understood. Here we reveal that phosphatidylinositol 3-kinase (PI3K) signalling is activated in response to peripheral axotomy and that PI3K pathway is required for sensory axon regeneration. Moreover, we show that glycogen synthase kinase 3 (GSK3), rather than mammalian target of rapamycin, mediates PI3K-dependent augmentation of the growth potential in the PNS. Furthermore, we show that PI3K–GSK3 signal is conveyed by the induction of a transcription factor Smad1 and that acute depletion of Smad1 in adult mice prevents axon regeneration in vivo . Together, these results suggest PI3K–GSK3–Smad1 signalling as a central module for promoting sensory axon regeneration in the mammalian nervous system. Mature neurons in the mammalian central nervous system (CNS) fail to regenerate axons after injury due to diminished intrinsic growth capacity coupled with the hostile CNS environment [1] , [2] , [3] , [4] . By contrast, neurons in the mammalian peripheral nervous system (PNS) regenerate axons, as neurons in most invertebrates, in part, by enhancing their intrinsic growth ability. The power of genetic approaches in relatively simple organisms, such as Caenorhabditis elegans or Drosophila , have greatly facilitated the investigation of components and pathways that are essential for axon regeneration in such model organisms [5] , [6] , [7] , [8] . The signalling pathways, however, triggered by peripheral axotomy that induces spontaneous axon regeneration in the mammalian nervous system remain poorly understood [9] . Peripheral nerve injury causes profound cellular responses. In the severed axon, cytoskeletal and membrane components undergo dynamic reorganization to reseal the damaged membrane and form an advancing growth cone [10] , [11] . In the axotomized neuronal cell body, synthesis of mRNAs and proteins takes place to re-programme the damaged neuron and support lengthy regeneration [12] , [13] , [14] . Multiple factors participate in these processes, but the repair process might be governed by critical node molecules or pathways that coordinate seemingly complex regenerative responses. In the distal axon, glycogen synthase kinase 3 (GSK3) appears to coordinate cytoskeletal reorganization by regulating microtubule assembly and dynamics [10] , [15] , [16] , properties which are essential for axon regeneration [10] , [16] , [17] , [18] . In addition to its role in local cytoskeletal dynamics, GSK3 is known to control gene transcription [19] , [20] by regulating the activities of a myriad of transcription factors [19] . Many such transcription factors, such as c-Jun, CREB and Smad, have been implicated in nerve injury and/or axonal repair [21] , [22] , [23] , but whether GSK3 has a role in axon regeneration through inducing transcriptional responses remains unknown. Adult mouse dorsal root ganglion (DRG) neurons represent a favourable system to study mammalian axon regeneration. Each DRG neuron develops an axon that bifurcates into a central branch entering the CNS and a peripheral branch innervating sensory targets. In contrast to the central branch that fails to regrow after injury, axotomy of the peripheral branch often induces successful axon regeneration. In fact, an injury at the peripheral branch, known as a ‘conditioning lesion’, can prime sensory neurons into an active growth state and dramatically increase regenerative response to a second lesion occurring at either the peripheral or the central branch [24] , [25] , [26] , [27] , [28] . Previous work has suggested that this enhanced growth state requires activation of transcription-dependent proregenerative signalling, which might trigger the expression of a number of regeneration-associated genes (RAGs) [13] . It is likely that post-traumatic signals induced by peripheral axotomy regulate key transcription factors, which in turn would control the expression of downstream targets. Although several factors have been implicated in mammalian axon regeneration, little is known about the interplay among such molecules and the signalling pathway leading to the activation of proregenerative transcriptional programme. The present study shows that peripheral nerve injury activates phosphatidylinositol 3-kinase (PI3K) signalling, leading to inactivation of GSK3. In contrast to CNS regeneration [29] , we find that mammalian target of rapamycin (mTOR) is dispensable for sensory axon regeneration. Instead, GSK3 conveys PI3K signalling in the PNS by inducing the expression of a transcription factor smad1 . Furthermore, acutely blocking PI3K signalling or depleting Smad1 in adult mice prevents sensory axon regeneration in vivo , suggesting PI3K–GSK3–Smad1 pathway as a critical module that induces spontaneous axon regeneration in the mammalian nervous system. Establishing an in vitro model for axon regeneration To investigate signalling components or pathways involved in axon regeneration, we established an in vitro model ( Fig. 1a ) that can recapitulate in vivo axon regeneration induced by peripheral axotomy. Similar to the induction of RAGs that occurs in vivo after peripheral axotomy, we detected a marked upregulation of several proteins encoded by well-known RAGs, such as gap43, c-jun, atf3 , gadd45α and sprr1a , in adult DRG neurons within 3 days of culture ( Fig. 1b ). When the cultured neurons were replated, neurons extended new axons that were long but sparsely branched ( Fig. 1c ), reminiscent of the morphology of conditioning lesioned neurons [28] . This elongating mode of axon growth is distinct from axon growth induced by nerve growth factor (NGF), which promotes extensive branching, but relatively modest lengthening in adult DRG neurons ( Fig. 1c ). These results show that adult DRG neurons acquire biochemical and morphological properties similar to pre-conditionally injured neurons after undergoing culture-and-replating procedures. 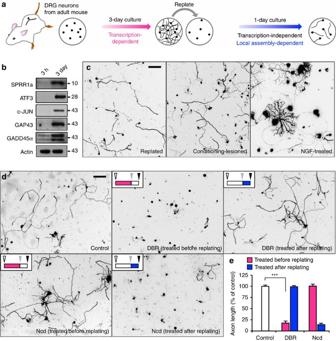Figure 1: Establishment of a culture-and-replate protocol to investigate mechanisms of regenerative axon growthin vitro. (a) Schematics of the culture-and-replate protocol. DRG neurons were dissociated from adult mice and cultured for 3 days. Neurons were then replated to initiate axon growth anew. Regenerative axon growth was assessed by measuring axon length from replated neurons at 20 h after replating. (b)In vitroculture recapitulates peripheral axotomy-induced upregulation of several proteins that are encoded by well-known RAGs such as ATF3, c-Jun, GAP43, GADD45a and SPRR1a. Shown are representative immunoblots from DRG neuronal lysates cultured for either 3 h or 3 days. Actin antibodies were used as a loading control. (c) DRG neurons grow long, sparsely branched axons after replating, similar to neurons that were conditionedin vivoby sciatic nerve transection. Note that the mode of axon growth after replating is distinct from that induced by NGF (50 ng ml−1), which stimulates extensive branching but relatively modest lengthening. Scale bar, 200 μm. (d,e) Adult DRG neurons were dissociated, cultured for 3 days and then replated to induce axon growth anew, as depicted ina. Neurons were treated with DBR (20 μM), nocodazole (50 nM) or vehicle control (DMSO) either before (magenta bars ine) or after replating (blue bars ine), as indicated. Schematics (upper left insets ind) depict when the neurons were treated with drugs of interest. Coloured bars indicate the period when neurons were exposed to drugs. White, grey and black arrowheads indicate the starting point of the initial 3-day-culture period, the time of replating and when neurons were fixed for the analysis, respectively. Regenerative axon growth was assessed by measuring axon length after replating. Representative images neurons after replating are shown ind. Quantification of axon length from three independent experiments is shown ine. Scale bar, 200 μm. Error bars represent s.e.m. ***P<0.001, unpaired two-tailed Student’st-test. Original immunoblot images are shown inSupplementary Fig. S10. Figure 1: Establishment of a culture-and-replate protocol to investigate mechanisms of regenerative axon growth in vitro . ( a ) Schematics of the culture-and-replate protocol. DRG neurons were dissociated from adult mice and cultured for 3 days. Neurons were then replated to initiate axon growth anew. Regenerative axon growth was assessed by measuring axon length from replated neurons at 20 h after replating. ( b ) In vitro culture recapitulates peripheral axotomy-induced upregulation of several proteins that are encoded by well-known RAGs such as ATF3, c-Jun, GAP43, GADD45a and SPRR1a. Shown are representative immunoblots from DRG neuronal lysates cultured for either 3 h or 3 days. Actin antibodies were used as a loading control. ( c ) DRG neurons grow long, sparsely branched axons after replating, similar to neurons that were conditioned in vivo by sciatic nerve transection. Note that the mode of axon growth after replating is distinct from that induced by NGF (50 ng ml −1 ), which stimulates extensive branching but relatively modest lengthening. Scale bar, 200 μm. ( d , e ) Adult DRG neurons were dissociated, cultured for 3 days and then replated to induce axon growth anew, as depicted in a . Neurons were treated with DBR (20 μM), nocodazole (50 nM) or vehicle control (DMSO) either before (magenta bars in e ) or after replating (blue bars in e ), as indicated. Schematics (upper left insets in d ) depict when the neurons were treated with drugs of interest. Coloured bars indicate the period when neurons were exposed to drugs. White, grey and black arrowheads indicate the starting point of the initial 3-day-culture period, the time of replating and when neurons were fixed for the analysis, respectively. Regenerative axon growth was assessed by measuring axon length after replating. Representative images neurons after replating are shown in d . Quantification of axon length from three independent experiments is shown in e . Scale bar, 200 μm. Error bars represent s.e.m. *** P <0.001, unpaired two-tailed Student’s t -test. Original immunoblot images are shown in Supplementary Fig. S10 . Full size image We applied the culture-and-replating method to investigate whether regenerative axon growth requires gene transcription. For this purpose, a reversible inhibitor of RNA polymerase II, 5,6-dichlorobenzimidazole riboside (DBR), was treated. As expected, adding DBR during the initial 3-day-culture period nearly abolished axon growth ( Supplementary Fig. S1 ), suggesting the requirement of gene transcription. Neurons treated with DBR during the initial 3-day-culture period failed to grow axons after replating, even when DBR was washed out at the time of replating, and then the neurons were cultured without the drug thereafter ( Fig. 1d,e ). These results suggest that gene transcription during the initial 3-day-culture period is essential for both the initial and regenerative axon growth. By contrast, when neurons were first cultured in the absence of DBR, but DBR was added at the time of replating and thereafter, replated neurons extended axons to an extent comparable to control neurons that were never exposed to DBR ( Fig. 1d,e ). These results are consistent with the previous study showing that DBR did not affect axon growth in culture if neurons had been pre-conditioned in vivo several days prior to the dissociation [28] . Therefore, a discrete period of active gene transcription is essential for mature neurons to gain growth competence and once neurons have undergone this process, axon extension can occur without on-going transcription. Along with gene transcription, microtubule assembly in the distal axon is another crucial determinant of axon regeneration [10] , [17] , [18] , [30] . As expected, dampening microtubule dynamics by treating nocodazole during the initial 3-day-culture period drastically prevented axon growth ( Supplementary Fig. S1 ). However, replated neurons extended long axons when nocodazole was washed out at the time of replating ( Fig. 1d,e ), starkly contrasting with the results from DBR-treatment. When neurons were first cultured in the absence of nocodazole, but treated with the drug at the time of replating and thereafter, replated neurons failed to extend axons ( Fig. 1d,e ), again showing completely opposite results from DBR-treatment. In summary, the culture-and-replating protocol described here recapitulates biochemical ( Fig. 1b ) and morphological properties ( Fig. 1c ) of axon regeneration triggered by nerve injury, and provides an experimentally accessible system to investigate transcription-dependent and local assembly dependent mechanisms of axon growth. Intrinsic axon growth ability is acquired by PI3K signalling Using the culture-and-replating protocol, we searched for potential regulators of axon regeneration by applying selective inhibitors against known signalling molecules. We found that LY294002, an inhibitor of PI3K, inhibited regenerative axon growth when it was applied before but not after replating ( Fig. 2a,b ). U0126, an inhibitor of the ERK pathway, had little effect regardless of the time of drug treatment ( Fig. 2a,b ). In addition to affecting axon length, LY294002 increased the frequency of axonal branching without altering total number of branches ( Supplementary Fig. S2 ). LY294002 inhibited axon growth in bax −/− neurons to an extent similar to wild type ( Fig. 2c ), excluding the possibility that impaired axon growth occurs as a secondary consequence of diminished cell viability. Confirming pharmacological data, axon growth was inhibited by expressing a dominant-negative construct of PI3K (dnPI3K) ( Fig. 2d–f ), which effectively blocked PI3K signalling, as evidenced by suppression of AKT phosphorylation ( Fig. 2d ). Together, these results suggest PI3K signalling as a potential regulator of axon regeneration. 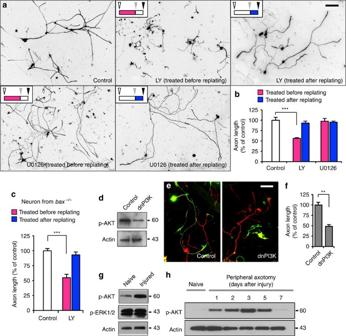Figure 2: Activation of PI3K signalling is essential for augmentation of axon growth potential. (a,b) Adult DRG neurons were cultured as depicted inFig. 1a. Neurons were treated with LY294002 (LY, 10 μM), U0126 (20 μM) or vehicle control (DMSO) either before (magenta bars inb) or after replating (blue bars inb), as indicated. Regenerative axon growth was assessed by measuring axon length after replating. Representative images of replated neurons are shown ina. Quantification of axon length from three independent experiments is shown inb. Scale bar, 200 μm. Error bars represent s.e.m. ***P<0.001, unpaired two-tailed Student’st-test. (c) Adult DRG neurons frombax−/−mice were cultured as depicted inFig. 1a. Neurons were treated with LY294002 (LY, 10 μM) or vehicle control (DMSO) either before (magenta bar) or after replating (blue bar), as indicated. Regenerative axon growth was assessed by measuring axon length after replating. Quantification of axon length from three independent experiments is shown. Error bars represent s.e.m. ***P<0.001, unpaired two-tailed Student’st-test. (d) Validation of the dominant-negative PI3K construct (dnPI3K). Representative immunoblots from 3-day-cultured DRG neurons transfected with either dnPI3K or a control vector (EGFP). (e,f) Dissociated adult DRG neurons were transfectedin vitrowith EGFP alone (control) or with dnPI3K (myc tagged). Neurons were cultured for 3 days, followed by replating to initiate axon growth anew. Neurons were fixed at 20 h after replating and stained for neuronal tubulin βIII, TuJ1 (red) or the myc tag. Transfected neurons are shown in green (EGFP or myc positive neurons). Representative images of replated neurons are shown ine. Quantification of axon length from three independent experiments is shown inf. Scale bar, 100 μm. Error bars represent s.e.m. **P<0.01, unpaired two-tailed Student’st-test. (g) Representative immunoblots of phosphorylated Akt and ERK1/2 detected in DRGs from naive or injured mice that were subjected to sciatic nerve transection. (h) Representative immunoblots of time-course analysis of AKT phosphorylation in DRGs in response to peripheral nerve injury. Original immunoblot images are shown inSupplementary Fig. S10. Figure 2: Activation of PI3K signalling is essential for augmentation of axon growth potential. ( a , b ) Adult DRG neurons were cultured as depicted in Fig. 1a . Neurons were treated with LY294002 (LY, 10 μM), U0126 (20 μM) or vehicle control (DMSO) either before (magenta bars in b ) or after replating (blue bars in b ), as indicated. Regenerative axon growth was assessed by measuring axon length after replating. Representative images of replated neurons are shown in a . Quantification of axon length from three independent experiments is shown in b . Scale bar, 200 μm. Error bars represent s.e.m. *** P <0.001, unpaired two-tailed Student’s t -test. ( c ) Adult DRG neurons from bax −/− mice were cultured as depicted in Fig. 1a . Neurons were treated with LY294002 (LY, 10 μM) or vehicle control (DMSO) either before (magenta bar) or after replating (blue bar), as indicated. Regenerative axon growth was assessed by measuring axon length after replating. Quantification of axon length from three independent experiments is shown. Error bars represent s.e.m. *** P <0.001, unpaired two-tailed Student’s t -test. ( d ) Validation of the dominant-negative PI3K construct (dnPI3K). Representative immunoblots from 3-day-cultured DRG neurons transfected with either dnPI3K or a control vector (EGFP). ( e , f ) Dissociated adult DRG neurons were transfected in vitro with EGFP alone (control) or with dnPI3K (myc tagged). Neurons were cultured for 3 days, followed by replating to initiate axon growth anew. Neurons were fixed at 20 h after replating and stained for neuronal tubulin βIII, TuJ1 (red) or the myc tag. Transfected neurons are shown in green (EGFP or myc positive neurons). Representative images of replated neurons are shown in e . Quantification of axon length from three independent experiments is shown in f . Scale bar, 100 μm. Error bars represent s.e.m. ** P <0.01, unpaired two-tailed Student’s t -test. ( g ) Representative immunoblots of phosphorylated Akt and ERK1/2 detected in DRGs from naive or injured mice that were subjected to sciatic nerve transection. ( h ) Representative immunoblots of time-course analysis of AKT phosphorylation in DRGs in response to peripheral nerve injury. Original immunoblot images are shown in Supplementary Fig. S10 . Full size image We observed that the level of phospho-AKT but not that of phospho-ERK increased in response to peripheral nerve transection ( Fig. 2g ). Detailed time-course analysis revealed that phosphorylation of AKT peaked at 3 days, followed by dephosphorylation to baseline levels after 7 days ( Fig. 2h ), suggesting activation of PI3K signalling. When we acutely blocked PI3K signalling prior to sciatic nerve injury by transfecting dnPI3K into adult DRGs by in vivo electroporation, sensory axon regeneration was substantially impaired ( Fig. 3b,c , Supplementary Fig. S7 ). These results demonstrate that PI3K signalling is required specifically in the mature nervous system for enhancing axon regeneration. 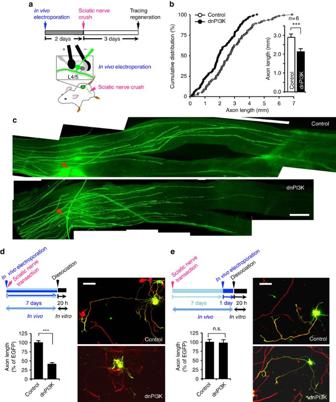Figure 3: PI3K signalling is required for activating proregenerative responses and subsequent axon regenerationin vivo. (a) Schematics ofin vivoelectroporation and investigation of axon regeneration. (b,c) L4/ L5 DRGs of an adult mouse were electroporatedin vivowith EGFP alone (control) or together with dominant-negative PI3K (dnPI3K) at a ratio of 1:3, followed by the sciatic nerve crush as depicted ina. The lengths of all identifiable regenerating axons in the whole-mount nerves were measured from the crush site (arrowheads) to the distal axon tips. Lengths of total of 120 axons from six control mice and 124 axons from six dnPI3K-transfected mice were measured. Quantification of axon length is shown inband representative images are shown inc. Scale bar, 500 μm. Error bars represent s.e.m. ***P<0.00001, unpaired two-tailed Student’st-test. (d) L4/L5 DRGs in adult mice were electroporatedin vivowith EGFP (control) or dnPI3K (myc-tagged), immediately followed by sciatic nerve transection. At 7 days after sciatic nerve transection, neurons from L4/L5 DRGs were cultured overnight and stained for neuronal tubulin, TuJ1 (red) or the myc tag. Transfected neurons are shown in green (EGFP or the myc positive). Experimental scheme is depicted in the upper left. Representative images (right) and quantification of axon length (lower left) from three independent experiments are shown. Scale bar, 100 μm. Error bars represent s.e.m. ***P<0.001, unpaired two-tailed Student’st-test. (e) Adult mice were first subjected to sciatic nerve transection. At 7 days after the nerve injury, L4/L5 DRGs were electroporatedin vivowith EGFP (control) or dnPI3K (myc tagged). One day after thein vivoelectroporation, neurons from L4/L5 DRGs were cultured overnight and stained for neuronal tubulin, TuJ1 (red) or the myc tag. Transfected neurons are shown in green (EGFP or the myc positive). Experimental scheme is depicted in the upper left. Representative images (right) and quantification of axon length (lower left) from three independent experiments are shown. Scale bar, 100 μm. Error bars represents s.e.m. ***P<0.001, unpaired two-tailed Student’st-test. Figure 3: PI3K signalling is required for activating proregenerative responses and subsequent axon regeneration in vivo . ( a ) Schematics of in vivo electroporation and investigation of axon regeneration. ( b , c ) L4/ L5 DRGs of an adult mouse were electroporated in vivo with EGFP alone (control) or together with dominant-negative PI3K (dnPI3K) at a ratio of 1:3, followed by the sciatic nerve crush as depicted in a . The lengths of all identifiable regenerating axons in the whole-mount nerves were measured from the crush site (arrowheads) to the distal axon tips. Lengths of total of 120 axons from six control mice and 124 axons from six dnPI3K-transfected mice were measured. Quantification of axon length is shown in b and representative images are shown in c . Scale bar, 500 μm. Error bars represent s.e.m. *** P <0.00001, unpaired two-tailed Student’s t -test. ( d ) L4/L5 DRGs in adult mice were electroporated in vivo with EGFP (control) or dnPI3K (myc-tagged), immediately followed by sciatic nerve transection. At 7 days after sciatic nerve transection, neurons from L4/L5 DRGs were cultured overnight and stained for neuronal tubulin, TuJ1 (red) or the myc tag. Transfected neurons are shown in green (EGFP or the myc positive). Experimental scheme is depicted in the upper left. Representative images (right) and quantification of axon length (lower left) from three independent experiments are shown. Scale bar, 100 μm. Error bars represent s.e.m. *** P <0.001, unpaired two-tailed Student’s t -test. ( e ) Adult mice were first subjected to sciatic nerve transection. At 7 days after the nerve injury, L4/L5 DRGs were electroporated in vivo with EGFP (control) or dnPI3K (myc tagged). One day after the in vivo electroporation, neurons from L4/L5 DRGs were cultured overnight and stained for neuronal tubulin, TuJ1 (red) or the myc tag. Transfected neurons are shown in green (EGFP or the myc positive). Experimental scheme is depicted in the upper left. Representative images (right) and quantification of axon length (lower left) from three independent experiments are shown. Scale bar, 100 μm. Error bars represents s.e.m. *** P <0.001, unpaired two-tailed Student’s t -test. Full size image To investigate when PI3K signalling has a role, we interfered with PI3K signalling either before or after the onset of proregenerative responses and examined the consequences on axon growth. When in vivo electroporation of dnPI3K was performed right before sciatic nerve transection and then neurons from the transfected DRGs were cultured 7 days later ( Fig. 3d ), dnPI3K-transfected neurons extended shorter axons compared with control neurons transfected with EGFP prior to peripheral axotomy ( Fig. 3d ). By contrast, dnPI3K failed to block axon growth when in vivo electroporation was performed 7 days after nerve transection ( Fig. 3e ). Together, these results provide ample evidence that PI3K pathway should be activated prior to augmentation of the transcription-dependent regenerative programme to promote axon regeneration. GSK3 rather than mTOR conveys PI3K signalling Depletion of pten ( phosphatase and tensin homolog ), a gene encoding a phosphatase that directly counteracts the activity of PI3K, could promote axon regeneration both in CNS [29] and PNS [31] . In CNS, activation of mTOR, a well-known regulator of protein translation [32] , has been suggested to mediate the growth-promoting effect of pten depletion [29] , [33] . In PNS, involvement of mTOR has been investigated, yielding seemingly controversial results. One study suggested that mTOR signalling is dispensable for enhancing axon regeneration induced by PTEN inhibition [31] , whereas another study has shown that inhibition of mTOR suppressed axon growth in adult DRG neurons [34] . The apparent discrepancy might be attributed to different culture conditions such as application of growth factors. Indeed, the latter study applied a high concentration of NGF, which is known to activate a number of signalling pathways and therefore might complicate the interpretation of data. In our condition, neurons were cultured without adding NGF or any other growth factors. In this condition, rapamycin failed to inhibit axon growth regardless of the time of drug treatment ( Fig. 4a,b ). We confirmed that rapamycin treatment completely prevented phosphorylation of S6 ( Fig. 4c,d ), a downstream effector of mTOR, and thus could rule out the involvement of mTOR in regulating regenerative axon growth from adult DRG neurons. By contrast, application of cycloheximide, a general inhibitor of protein translation, either before or after replating nearly abolished axon growth ( Fig. 4a,b ). These results suggest that PI3K signalling promotes axon regeneration in an mTOR-independent fashion in adult sensory neurons. 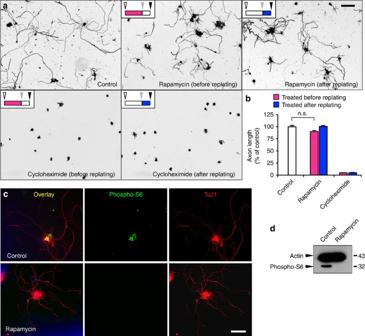Figure 4: Regenerative axon growth from adult sensory neurons requires mTOR-independent protein synthesis. (a,b) Adult DRG neurons were dissociated, cultured for 3 days and then replated to initiate axon growth anew, as depicted inFig. 1a. Neurons were treated with rapamycin (20 nM), cycloheximide (5 μg ml−1) or DMSO (control) either before (magenta bars inb) or after replating (blue bars inb), as indicated, and axon length was measured at 20 h after replating. The schematics and symbols (upper left insets ina) are identical toFig. 1d. Representative images of replated neurons are shown inaand quantification of axon length from three independent experiments is shown inb. Scale bar, 200 μm. Error bars represent s.e.m. n.s., statistically insignificant difference, unpaired two-tailed Student’st-test. (c) Representative images of control (upper panels) and rapamycin-treated (lower panels) adult DRG neurons immunostained with TuJ1 and phospho-S6 antibodies. Note that rapamycin treatment completely prevented S6 phosphorylation but had no effect on axon growth. Scale bar, 200 μm. (d) Representative immunoblots from adult DRG neurons cultured for 3 days in the presence or absence of rapamycin. Actin antibodies were used as a loading control. Note that rapamycin treatment completely prevented S6 phosphorylation. Original immunoblot image is shown inSupplementary Fig. S11. Figure 4: Regenerative axon growth from adult sensory neurons requires mTOR-independent protein synthesis. ( a , b ) Adult DRG neurons were dissociated, cultured for 3 days and then replated to initiate axon growth anew, as depicted in Fig. 1a . Neurons were treated with rapamycin (20 nM), cycloheximide (5 μg ml −1 ) or DMSO (control) either before (magenta bars in b ) or after replating (blue bars in b ), as indicated, and axon length was measured at 20 h after replating. The schematics and symbols (upper left insets in a ) are identical to Fig. 1d . Representative images of replated neurons are shown in a and quantification of axon length from three independent experiments is shown in b . Scale bar, 200 μm. Error bars represent s.e.m. n.s., statistically insignificant difference, unpaired two-tailed Student’s t -test. ( c ) Representative images of control (upper panels) and rapamycin-treated (lower panels) adult DRG neurons immunostained with TuJ1 and phospho-S6 antibodies. Note that rapamycin treatment completely prevented S6 phosphorylation but had no effect on axon growth. Scale bar, 200 μm. ( d ) Representative immunoblots from adult DRG neurons cultured for 3 days in the presence or absence of rapamycin. Actin antibodies were used as a loading control. Note that rapamycin treatment completely prevented S6 phosphorylation. Original immunoblot image is shown in Supplementary Fig. S11 . Full size image GSK3s represent alternative targets of PI3K signalling and have prominent roles in axon growth [20] . We detected a marked increase in the N-terminal serine phosphorylations of GSK3s (phospho-Ser9-GSK3β; phospho-Ser21-GSK3a) and a concomitant decrease in GSK3-dependent phosphorylation of CRMP2 in response to sciatic nerve transection ( Fig. 5a ), suggestive of their inactivation. Increase in Ser9-GSK3 phosphorylation that occurred in vivo ( Fig. 5a ) was recapitulated in vitro ( Fig. 5b ), which was nearly abolished by LY294002, placing GSK3 downstream of PI3K signalling. Moreover, axonal elongation defect induced by PI3K inhibition was completely rescued by applying two different inhibitors of GSK3, 6-bromoindirubin-3′-acetoxime (BIO) or SB216763 ( Fig. 5c,d ). Notably, GSK3 inhibitors rescued LY294002-induced axonal elongation defect, only when applied before replating, followed by washout at the time of replating. By contrast, BIO substantially blocked axon growth when treated after replating ( Supplementary Fig. S3 ), an effect which is in line with our previous study suggesting that depletion of GSK3 prevents local axon assembly in the growth cone [16] . These results suggest that inhibition of GSK3 in the soma and the distal axon produces opposite effects. 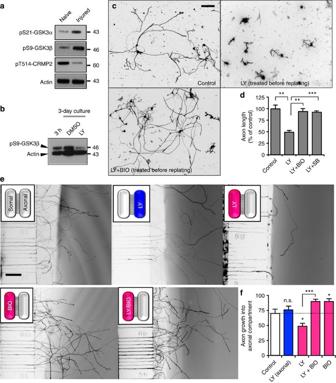Figure 5: Inactivation of GSK3 in the cell body is responsible for augmentation of transcription-dependent axon growth potential downstream of PI3K signalling. (a) Representative immunoblots of phosphorylated GSK3α-Ser21, GSK3β-Ser9 and CRMP2-Thr514 detected in L4/5 DRG lysates from naïve or injured mice that were subjected to sciatic nerve transection. (b) Representative immunoblots of phosphorylated GSK3β-Ser9 detected in dissociated adult DRG neurons cultured for either 3 h or 3 days. For the 3-day cultures, neurons were treated with LY294002 (LY, 10 μM) or vehicle control (DMSO), as indicated. (c,d) Adult DRG neurons were dissociated, cultured for 3 days and then replated. Neurons were treated with 6-bromoindirubin-3′-acetoxime (BIO, 500 nM), SB216763 (SB, 10 μM) and/or LY294002 (LY, 10 μM), as indicated, during the initial 3-day-culture period. Replated neurons were cultured in the absence of drugs. Axon length was measured at 20 h after replating. Representative images of replated neurons are shown incand quantification of axon length from three independent experiments is shown ind. Scale bar, 200 μm. Error bars represent s.e.m.**P<0.01; ***P<0.001, unpaired two-tailed Student’st-test. (e,f) Adult DRG neurons were loaded in the somal side of the two-compartment chambers as described in Methods. LY294002 (LY, 10 μM) and/or BIO (500 nM, GSK3i) was locally applied either in the somal (magenta bars inf) or the axonal side (blue bar inf), as indicated.yaxis infdepicts the number of microchannels occupied by axons exiting the channels and entering the axonal side (after normalization against the total number of channels). Representative images (e) and quantification (f) of axons entering the axonal compartment are shown. Schematics of the two-compartment chambers (upper left corner) depict where drugs were added. Treatment to the axonal and the somal side is illustrated in blue and magenta, respectively. Scale bar, 200 μm.n=3, error bars represent s.e.m. *P<0.01 compared with control; ***P<0.001; n.s. statistically insignificant difference compared to control, unpaired two-tailed Student’st-test. Original immunoblot images are shown inSupplementary Fig. S11. Figure 5: Inactivation of GSK3 in the cell body is responsible for augmentation of transcription-dependent axon growth potential downstream of PI3K signalling. ( a ) Representative immunoblots of phosphorylated GSK3α-Ser21, GSK3β-Ser9 and CRMP2-Thr514 detected in L4/5 DRG lysates from naïve or injured mice that were subjected to sciatic nerve transection. ( b ) Representative immunoblots of phosphorylated GSK3β-Ser9 detected in dissociated adult DRG neurons cultured for either 3 h or 3 days. For the 3-day cultures, neurons were treated with LY294002 (LY, 10 μM) or vehicle control (DMSO), as indicated. ( c , d ) Adult DRG neurons were dissociated, cultured for 3 days and then replated. Neurons were treated with 6-bromoindirubin-3′-acetoxime (BIO, 500 nM), SB216763 (SB, 10 μM) and/or LY294002 (LY, 10 μM), as indicated, during the initial 3-day-culture period. Replated neurons were cultured in the absence of drugs. Axon length was measured at 20 h after replating. Representative images of replated neurons are shown in c and quantification of axon length from three independent experiments is shown in d . Scale bar, 200 μm. Error bars represent s.e.m. ** P <0.01; *** P <0.001, unpaired two-tailed Student’s t -test. ( e , f ) Adult DRG neurons were loaded in the somal side of the two-compartment chambers as described in Methods. LY294002 (LY, 10 μM) and/or BIO (500 nM, GSK3i) was locally applied either in the somal (magenta bars in f ) or the axonal side (blue bar in f ), as indicated. y axis in f depicts the number of microchannels occupied by axons exiting the channels and entering the axonal side (after normalization against the total number of channels). Representative images ( e ) and quantification ( f ) of axons entering the axonal compartment are shown. Schematics of the two-compartment chambers (upper left corner) depict where drugs were added. Treatment to the axonal and the somal side is illustrated in blue and magenta, respectively. Scale bar, 200 μm. n =3, error bars represent s.e.m. * P <0.01 compared with control; *** P <0.001; n.s. statistically insignificant difference compared to control, unpaired two-tailed Student’s t -test. Original immunoblot images are shown in Supplementary Fig. S11 . Full size image To further investigate differing roles of the PI3K–GSK3 signalling in the regulation of cell body- versus local assembly dependent mechanisms, we utilized two-compartment culture platforms that permit fluidic isolation of somal and axonal compartments [30] , [35] . Consistent with the culture-and-replating experiments ( Fig. 2a,b ), LY294002 blocked axon growth only when treated into the somal but not the axonal side ( Fig. 5e,f ). Local administration of BIO into the somal compartment completely rescued the impaired axon growth induced by LY294002 ( Fig. 4e,f ), supporting the notion that PI3K–GSK3 pathway regulates axon regeneration by controlling cell body responses (that is, transcription-dependent augmentation of intrinsic axon growth potential), rather than regulating axonal responses. In the culture-and-replating experiment, treatment of BIO alone before replating induced a small but statistically significant enhancement of axon growth compared with control (~15% increase) ( Supplementary Fig. S3 ). Consistently, applying BIO alone in the somal compartment enhanced axon growth (by ~28%) ( Fig. 5e,f ), demonstrating a discernable growth-promoting effect. Nonetheless, in both the culture-and-replating and the two-compartment chamber experiments, axon growth defect caused by PI3K inhibition was fully rescued by GSK3 inactivation ( Fig. 5d,f ), suggesting that GSK3 in the cell body functions specifically downstream of PI3K to control axon growth, although somal inactivation of GSK3 exerts some general growth-augmenting effect. β-catenin is dispensable for sensory axon regeneration Next, we searched for a downstream effector of the PI3K–GSK3 pathway that might be responsible for the cell body response. For this purpose, we tested the possible involvement of β-catenin, a well-known substrate of GSK3 and a regulator of gene transcription. However, neither peripheral nerve injury ( Fig. 6a ) nor blockade of PI3K signalling ( Fig. 6b ) altered the level of β-catenin. Furthermore, depletion of β-catenin had no effect on axon regeneration in vivo ( Fig. 6c–e , Supplementary Fig. S8 ), excluding the involvement of β-catenin in sensory axon regeneration. 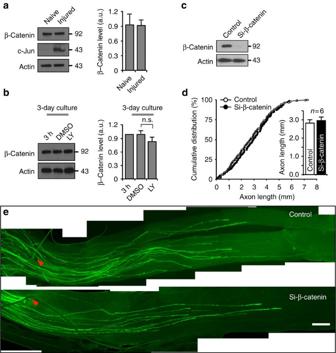Figure 6: β-catenin is dispensable for sensory axon regeneration. (a) Representative immunoblots of DRG lysates from naive or injured mice. To induce injury, mice were subjected to sciatic nerve transection and DRGs were collected after 3 days. Actin antibodies were used as a loading control. Quantification of β-catenin level normalized against actin is presented (right). (b) Representative immunoblots from DRG neurons cultured for either 3 h or 3 days. For the 3 day cultures, neurons were grown in the presence of LY294002 (LY, 10 μM) or vehicle control (DMSO), as indicated. Actin antibodies were used as a loading control. Quantification of β-catenin level normalized against actin is presented (right). Error bars represent s.e.m. n.s., statistically insignificant difference, unpaired two-tailed Student’st-test. (c) Representative blots for validating the efficacy of the siRNA against β-catenin (si-β-catenin) afterin vivoelectroporation into DRGs. Actin antibodies were used as a loading control. (d,e) L4 and L5 DRGs of an adult mouse were electroporatedin vivowith either EGFP alone (control) or together with si-β-catenin, followed by sciatic nerve crush at 2 days after the electroporation. Axon regeneration was assessed by whole-mount analysis at 3 days after nerve injury.In vivoelectroporation and investigation of axon regeneration were performed as depicted inFig. 3a. Using whole-mount nerve segments, the lengths of all identifiable regenerating axons were measured from the crush site (arrowheads) to the distal axon tips. For quantification, lengths of a total of 145 axons from six control mice and 140 axons from six si-β-catenin-transfected mice were measured. Quantification (d) and representative images of axon regeneration (e) are shown. Scale bar, 500 μm. Error bars represent s.e.m. Original immunoblot images are shown inSupplementary Fig. S11. Figure 6: β-catenin is dispensable for sensory axon regeneration. ( a ) Representative immunoblots of DRG lysates from naive or injured mice. To induce injury, mice were subjected to sciatic nerve transection and DRGs were collected after 3 days. Actin antibodies were used as a loading control. Quantification of β-catenin level normalized against actin is presented (right). ( b ) Representative immunoblots from DRG neurons cultured for either 3 h or 3 days. For the 3 day cultures, neurons were grown in the presence of LY294002 (LY, 10 μM) or vehicle control (DMSO), as indicated. Actin antibodies were used as a loading control. Quantification of β-catenin level normalized against actin is presented (right). Error bars represent s.e.m. n.s., statistically insignificant difference, unpaired two-tailed Student’s t -test. ( c ) Representative blots for validating the efficacy of the siRNA against β-catenin (si-β-catenin) after in vivo electroporation into DRGs. Actin antibodies were used as a loading control. ( d , e ) L4 and L5 DRGs of an adult mouse were electroporated in vivo with either EGFP alone (control) or together with si-β-catenin, followed by sciatic nerve crush at 2 days after the electroporation. Axon regeneration was assessed by whole-mount analysis at 3 days after nerve injury. In vivo electroporation and investigation of axon regeneration were performed as depicted in Fig. 3a . Using whole-mount nerve segments, the lengths of all identifiable regenerating axons were measured from the crush site (arrowheads) to the distal axon tips. For quantification, lengths of a total of 145 axons from six control mice and 140 axons from six si-β-catenin-transfected mice were measured. Quantification ( d ) and representative images of axon regeneration ( e ) are shown. Scale bar, 500 μm. Error bars represent s.e.m. Original immunoblot images are shown in Supplementary Fig. S11 . Full size image Smad1 functions downstream of PI3K–GSK3 signalling Peripheral nerve injury could increase phosphorylation of a transcription factor Smad1 in the nucleus of DRG neurons, indicative of its activation [23] . Moreover, injection of bone morphogenetic protein (BMP) in vivo could increase Smad1 phosphorylation, accompanied by enhanced axon regeneration [36] , implying a role for Smad1 in axon regeneration. We observed increases in both phospho- and total-Smad1 after 3 days of culture, which were blocked by LY294002. We also observed that the LY294002-induced downregulation of Smad1 was fully rescued by BIO ( Fig. 7a,b ), suggesting Smad1 as a downstream target of PI3K–GSK3 signalling. As changes in phospho- and total-Smad1 occurred in parallel, we think that the rise and fall of phosphorylation occurs as a consequence of altered expression of Smad1, rather than through direct regulation of phosphorylation. 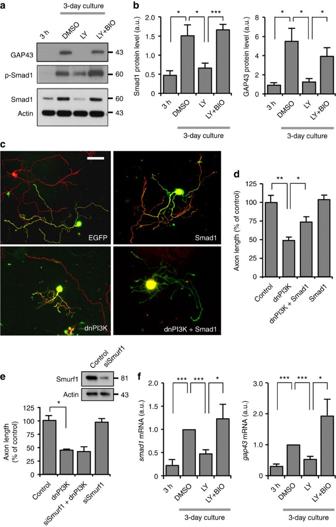Figure 7: Induction ofSmad1downstream of the PI3K–GSK3 pathway is essential for augmentation of the transcription-dependent axon growth potential. (a,b) Western blot analysis of DRG neurons cultured for 3 h or 3 days to examine the levels of phospho-Smad1 (p-Smad1), Smad1 or GAP43. For the 3 day cultures, neurons were treated with DMSO, LY294002 (LY, 10 μM) and/or 6-bromoindirubin-3′-acetoxime (BIO, 500 nM). Representative images and quantification of western blot analysis are shown inaandb.n=3, error bars represent s.e.m. *P<0.05; ***P<0.001, unpaired two-tailed Student’st-test. (c,d) Dissociated adult DRG neurons were transfectedin vitrowith EGFP, Smad1 (flag tagged) and/or dominant-negative PI3K (dnPI3K) (myc tagged). Neurons were cultured for 3 days and then replated for overnight culture. Neurons were then fixed and stained for neuronal tubulin, TuJ1, the flag tag or the myc tag. Representative images of replated neurons are shown incand quantification of axon length from three independent experiments is shown ind. Scale bar, 100 μm. Error bars represent s.e.m. *P<0.05; **P<0.001, unpaired two-tailed Student’st-test. (e) Dissociated adult DRG neurons were transfected with EGFP alone (control) or together with siRNAs against Smurf1 (siSmurf1) and/or dnPI3K, as indicated, and cultured for 3 days. Neurons were then replated and culture overnight. Quantification of axon length from three independent experiments is shown. Error bars represent s.e.m. *P<0.05, unpaired two-tailed Student’st-test. Efficacy of siSmurf1 was validated in adult DRG neurons (immunoblots in upper panel). (f) Adult DRG neurons cultured for 3 h or 3 days were subjected to qRT–PCR to examine the mRNA level ofsmad1orgap43. For the 3-day cultures, neurons were treated with DMSO, LY294002 (LY, 10 μM) and/or BIO (500 nM), as indicated. Values were normalized against the mRNA level of the DMSO-treated sample.n=3, error bars represent s.e.m. *P<0.05; ***P<0.001, unpaired two-tailed Student’st-test. Original immunoblot images are shown inSupplementary Fig. S12. Figure 7: Induction of Smad1 downstream of the PI3K–GSK3 pathway is essential for augmentation of the transcription-dependent axon growth potential. ( a , b ) Western blot analysis of DRG neurons cultured for 3 h or 3 days to examine the levels of phospho-Smad1 (p-Smad1), Smad1 or GAP43. For the 3 day cultures, neurons were treated with DMSO, LY294002 (LY, 10 μM) and/or 6-bromoindirubin-3′-acetoxime (BIO, 500 nM). Representative images and quantification of western blot analysis are shown in a and b . n =3, error bars represent s.e.m. * P <0.05; *** P <0.001, unpaired two-tailed Student’s t -test. ( c , d ) Dissociated adult DRG neurons were transfected in vitro with EGFP, Smad1 (flag tagged) and/or dominant-negative PI3K (dnPI3K) (myc tagged). Neurons were cultured for 3 days and then replated for overnight culture. Neurons were then fixed and stained for neuronal tubulin, TuJ1, the flag tag or the myc tag. Representative images of replated neurons are shown in c and quantification of axon length from three independent experiments is shown in d . Scale bar, 100 μm. Error bars represent s.e.m. * P <0.05; ** P <0.001, unpaired two-tailed Student’s t -test. ( e ) Dissociated adult DRG neurons were transfected with EGFP alone (control) or together with siRNAs against Smurf1 (siSmurf1) and/or dnPI3K, as indicated, and cultured for 3 days. Neurons were then replated and culture overnight. Quantification of axon length from three independent experiments is shown. Error bars represent s.e.m. * P <0.05, unpaired two-tailed Student’s t -test. Efficacy of siSmurf1 was validated in adult DRG neurons (immunoblots in upper panel). ( f ) Adult DRG neurons cultured for 3 h or 3 days were subjected to qRT–PCR to examine the mRNA level of smad1 or gap43 . For the 3-day cultures, neurons were treated with DMSO, LY294002 (LY, 10 μM) and/or BIO (500 nM), as indicated. Values were normalized against the mRNA level of the DMSO-treated sample. n =3, error bars represent s.e.m. * P <0.05; *** P <0.001, unpaired two-tailed Student’s t -test. Original immunoblot images are shown in Supplementary Fig. S12 . Full size image Notably, level of GAP43, which is often associated with potential for growth or axon regeneration, responded to manipulations of PI3K and GSK3 activities in a manner similar to Smad1 ( Fig. 7a,b ). To investigate the relevance of altered Smad1 expression in the regulation of axon growth, we examined whether overexpression of Smad1 could rescue the dnPI3K-induced axon growth inhibition. Ectopic expression of Smad1 was insufficient to promote axon growth on its own but reversed the dnPI3K-induced attenuation of axon growth ( Fig. 7c,d ), suggesting that Smad1 functions downstream of PI3K–GSK3 signalling to control axon growth. However, it should be noted that although the extent of rescue was substantial (~50%), the remaining 50% refractory to Smad1 overexpression clearly suggests the existence of additional downstream mediator(s) of PI3K signalling. To investigate the mechanism by which PI3K–GSK3 signalling controls Smad1, we examined the possible involvement of Smad-specific E3-ubiquitin protein ligase Smurf1. Previous literature suggested that phosphorylation of Smad1 by GSK3 marks Smad1 for Smurf1-dependent polyubiquitination and subsequent proteasomal degradation [37] , [38] , [39] . However, depletion of Smurf1 had no effect ( Fig. 7e ), excluding Smurf1-dependent proteasomal degradation as a mechanism to control the amount of Smad1 and subsequent axon growth. Instead, we found that mRNA level of Smad1 was regulated by PI3K–GSK3 signalling ( Fig. 7f ), suggesting gene transcription rather than protein stability as a mechanism to control Smad1 level. This transcriptional regulation of Smad1 is distinct from the well-entrenched post-translational regulation of Smad1, a mechanism exemplified in BMP signalling. BMP induces Smad1 phosphorylation and its subsequent translocation into the nucleus, where Smad1 controls gene expression [40] . As expected by the segregated activation pathways, BMP4 had no effect on AKT phosphorylation, and likewise, phospho- and total-Smad1 were unaffected by BIO ( Supplementary Fig. S4a,b ). In primed neurons, phospho-Smad1 was readily detected and localized almost exclusively in the nucleus, which was unaffected by BIO ( Supplementary Fig. S4c,d ). Transfection of dnPI3K prevented nuclear accumulation of phospho-Smad1 ( Supplementary Fig. S4c,d ), but this might be due to decreased expression of Smad1 (see Fig. 7 ). Collectively, these results suggest that PI3K–GSK3 signalling promotes axon regeneration by controlling Smad1, but through a mechanism distinct from BMP. As in the 3-day culture (see Fig. 7a ), peripheral axotomy increased both phospho- and total-Smad1 in DRGs ( Fig. 8a ). Importantly, transfection of siRNAs against Smad1 into adult DRGs substantially prevented sensory axon regeneration in vivo ( Fig. 8b,c , Supplementary Fig. S9 ). In vivo transfection of a phospho-mimetic form of Smad1, which is thought to be constitutively active [38] , was insufficient to mimic the preconditioning effect and failed to promote axon growth ( Supplementary Fig. S5 ). Together, these results suggest that Smad1 is required but not sufficient for inducing sensory axon regeneration. 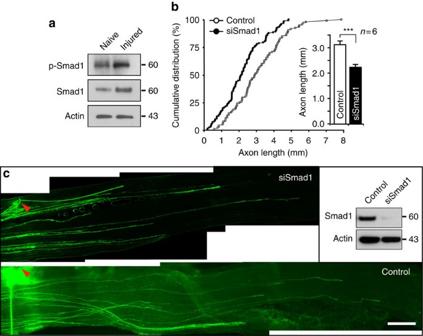Figure 8: Acute depletion of Smad1in vivoprevents sensory axon regeneration. (a) Representative immunoblots of DRG lysates from naive or injured mice. Mice were subjected to sciatic nerve transection to induce injury. DRGs were collected at 3 days after injury and subjected to western blot analysis. Representative immunoblots for phospho-Smad1 (p-Smad1) and Smad1 are shown. Actin antibodies were used as a loading control. (b,c) L4 and L5 DRGs of an adult mouse were electroporatedin vivowith either EGFP alone (control) or together with siRNAs against Smad1 (siSmad1), as indicated, followed by sciatic nerve crush at 2 days after the electroporation. Axon regeneration was assessed by whole-mount analysis at 3 days after nerve injury.In vivoelectroporation and investigation of axon regeneration were performed as depicted inFig. 3a. Using whole-mount nerve segments, the lengths of all identifiable regenerating axons were measured from the crush site (marked by epineural suture, arrowheads) to the distal axon tips. For quantification, lengths of a total of 92 axons from six control mice and 121 axons from six siSmad1-transfected mice were measured. Quantification (b) and representative images (c) of regenerating axons are shown. The inset shows knocking down of Smad1 by siSmad1 in adult DRG neuronsin vivo. Scale bar, 500 μm. Error bars represent s.e.m. *P<0.05, unpaired two-tailed Student’st-test. Original immunoblot images are shown inSupplementary Fig. S12. Figure 8: Acute depletion of Smad1 in vivo prevents sensory axon regeneration. ( a ) Representative immunoblots of DRG lysates from naive or injured mice. Mice were subjected to sciatic nerve transection to induce injury. DRGs were collected at 3 days after injury and subjected to western blot analysis. Representative immunoblots for phospho-Smad1 (p-Smad1) and Smad1 are shown. Actin antibodies were used as a loading control. ( b , c ) L4 and L5 DRGs of an adult mouse were electroporated in vivo with either EGFP alone (control) or together with siRNAs against Smad1 (siSmad1), as indicated, followed by sciatic nerve crush at 2 days after the electroporation. Axon regeneration was assessed by whole-mount analysis at 3 days after nerve injury. In vivo electroporation and investigation of axon regeneration were performed as depicted in Fig. 3a . Using whole-mount nerve segments, the lengths of all identifiable regenerating axons were measured from the crush site (marked by epineural suture, arrowheads) to the distal axon tips. For quantification, lengths of a total of 92 axons from six control mice and 121 axons from six siSmad1-transfected mice were measured. Quantification ( b ) and representative images ( c ) of regenerating axons are shown. The inset shows knocking down of Smad1 by siSmad1 in adult DRG neurons in vivo . Scale bar, 500 μm. Error bars represent s.e.m. * P <0.05, unpaired two-tailed Student’s t -test. Original immunoblot images are shown in Supplementary Fig. S12 . Full size image Axotomy-dependent downregulation of inositol phosphatases PI3K signalling is regulated by a balance between PI3K activity and the activities of inositol phosphatases that dephosphorylate PtdIns(3,4,5)P3. Thus, changes in the levels and/or activities of either PI3K or inositol phosphatases will shift the balance and affect the intensity and duration of PI3K signalling. Interestingly, we found that peripheral axotomy induced a substantial downregulation of several inositol phosphatases ( Supplementary Fig. S6 ), including pten , inpp4a , inpp4b and inpp5j , all of which encode negative regulators of AKT activation [41] , [42] , [43] . This result suggests that downregulation of inositol phosphatases in adult sensory neurons in response to peripheral axotomy might act upstream of the activation of PI3K signalling. The ability of PNS neurons to regenerate axons after nerve injury has been well documented for decades. Early work has suggested that a discrete period of gene transcription is essential for mature neurons to regain growth competence [28] , implying activation and/or induction of transcription factor(s) and co-factor(s) that can control the expression of a plethora of downstream target genes, and thereby mounting a cell-autonomous regenerative response. This study shows that peripheral axotomy activates PI3K–GSK3 signalling, which leads to the induction of Smad1, a key transcription factor for promoting axon regeneration in the mammalian nervous system. PI3K, GSK3 and Smad1 have critical roles in numerous cellular processes and their role in the nervous system, especially during development, has been the subject of intense investigation [20] , [44] , [45] , [46] . To investigate their roles specifically during axon regeneration in the mature nervous system, the present work applies in vivo electroporation, a technique that enables acute regulation of gene expression in the DRGs of adult mice, without inducing any compensatory responses during developmental stages [47] . By utilizing this method and varying the time of in vivo electroporation with respect to nerve injury, we could disrupt PI3K signalling in adult mice either right before or after the induction of proregenerative responses or acutely prevent the expression of Smad1, which would otherwise be induced by peripheral nerve injury. Through these experiments, this study provides compelling evidence that PI3K–Smad1 signalling promotes sensory axon regeneration specifically in the mature nervous system. However, further investigation is required to determine whether PI3K–Smad1 pathway is involved in enhancing the rate of axon regeneration or augmenting growth capacity in general. In vivo electroporation coupled with whole-mount analysis provides a way to directly trace entire paths of individual axons regenerating from the injury site to the distal tips. Despite this advantage, this approach is inappropriate for deducing any conclusion about the number of regenerating axons, because the number of EGFP-positive axons in our study reflects transfection efficiency (rather than growth potential), which varies substantially between animals. Moreover, in vivo electroporation affects only a small percentage of neurons, precluding functional or behavioural analysis. Introducing a kinase-inactivating mutation into one of the catalytic isoforms of PI3K (p110δ) was shown to inhibit axon regeneration and functional recovery following a sciatic nerve crush injury [48] , but the extent to which PI3K–GSK–Smad1 pathway contributes to functional recovery requires further investigation. The present study suggests that peripheral nerve injury turns on signalling downstream of PI3K activation, which has a crucial part in axon regeneration. PI3K generates phosphatidylinositol (3,4,5)-trisphosphate (PtdIns(3,4,5)P3), leading to a cascade of signalling events, including the recruitment and activation/inactivation of several kinases such as PDK1, AKT and GSK3. Here we show that peripheral axotomy induces activation of AKT ( Fig. 2g,h ) and inactivation of GSK3 ( Fig. 5a ) and that both events are sensitive to PI3K activity ( Figs 2d and 5b ). These results suggest that PI3K signalling is activated in response to peripheral injury, but there is no direct evidence for elevation of the kinase activity of PI3K per se . Inside a cell, level of PtdIns(3,4,5)P3, which controls the intensity and duration of PI3K signalling, is determined by the balance between its synthesis and degradation. Growth factor-receptor tyrosine kinase signalling is perhaps one of the best known pathways to elevate PtdIns(3,4,5)P3 by directly stimulating the kinase activity of PI3K. Theoretically, any alterations in the equilibrium between PI3K and inositol phosphatases that degrades PtdIns(3,4,5)P3 can readjust the level of PtdIns(3,4,5)P3 and affect subsequent signalling. Therefore, analogous to the regulatory mechanisms that directly alter the kinase activity of PI3K, modifications in the levels and/or activities of inositol phosphatases can shift the equilibrium and change inositol composition and subsequently control PI3K signalling. Indeed, peripheral axotomy induced a substantial downregulation of several inositol phosphatases ( Supplementary Fig. S6 ). It remains to be determined whether a shift in the balance of the phosphoinositide composition/turnover induced by peripheral nerve injury is sufficient to trigger the regenerative response or whether other receptor-mediated signalling induced by growth factors (or cytokines) secreted in an auto/paracrine fashion has a part. Together with our recent study [16] , our findings suggest GSK3 as a principal regulator of axon regeneration that coordinates regenerative responses in both soma and distal axons. On one hand, inhibition of GSK3 in the cell body enhances intrinsic growth competence by stimulating transcription-dependent axon regeneration programme. On the other hand, suppressing GSK3 activity to some extent in the growth cone promotes local cytoskeletal assembly by controlling microtubule dynamics. The extent of inactivation however should be controlled, as inhibition of GSK3 activity to a greater extent in the growth cone drastically blocks axon growth by preventing microtubule protrusion [10] , [16] . Although inactivation of GSK3 is important both in soma and distal axons, the two compartments might employ distinct regulatory mechanisms to achieve GSK3 inhibition. In the two-compartment cultures, application of LY294002 in the somal but not axonal compartment inhibited axon growth ( Fig. 4e,f ). Likewise, in the culture-and-replate experiments, regenerative axon growth was impaired only when LY294002 was treated before replating, but not after replating ( Fig. 2a,b ). In both experiments, axon growth defect induced by PI3K inhibition was fully reversed by inactivation of GSK3. These results suggest that PI3K controls GSK3 activity specifically in the soma to enhance growth competence, but is dispensable for local axon assembly in the distal axons. These mechanisms controlling sensory axon regeneration in adult neurons are in striking contrast to axon growth regulatory mechanisms in developing sensory neurons, where integrin signalling activates PI3K–GSK3 pathway specifically in the growth cone to control local axon assembly [49] . Upstream regulators responsible for modulating GSK3 signalling in growth cones of adult sensory neurons are yet to be defined. In response to peripheral axotomy, multiple pathways might contribute to bring about spontaneous axon regeneration. Induction of c-Jun in response to nerve injury has been well described [50] , and axon regeneration is severely compromised by depletion of c-Jun [47] . Whether c-Jun activation acts downstream of the PI3K signalling in regenerating neurons is currently unknown. In addition to functioning in neurons, recent studies suggest a role for c-Jun in the surrounding glial cells specialized for fostering axon regeneration and enhancing neuronal survival [51] , [52] . Spontaneous axon regeneration is therefore likely conferred by coordinated actions of multiple components and pathways functioning together in the complex injured environment. A more complete knowledge of the interplay among the pathways involved is warranted to advance our understanding of axon regeneration. Intriguingly, separate studies by different groups have independently shown that CNS regeneration in the mammalian nervous system could be promoted by directly manipulating each component of the PI3K–GSK3–Smad1 pathway: activation of PI3K signalling by genetic ablation of pten [33] , inactivation of GSK3 by administration of pharmacological inhibitors [53] or viral injection of BMP4 (an activator of Smad1 signalling) [36] could enhance CNS axon regeneration in rodent models of spinal cord injury. The finding that these molecules that have independently been identified to promote CNS axon regeneration are in fact interconnected as a signalling pathway in the PNS, where spontaneous regeneration occurs after injury, underscores the central role of the PI3K–GSK3–Smad1 module in regulating the growth potential and axon regeneration of mammalian neurons. Reagents LY294002, U0126, rapamycin and 6-bromoindirubin-3′-acetoxime (BIO) were from Calbiochem (San Diego, CA, USA). Dichlorobenzimidazole riboside (DBR) was from MP Biomedicals (Irvine, CA, USA). Cycloheximide and SB216763 were from Tocris Bioscience (Minneapolis, MN, USA). BMP4 was from PROSPEC (East Brunswick, NJ). The βIII tubulin (TuJ1), GAP43, c-myc and Flag antibodies were from Sigma-Aldrich. Antibodies against phospho-AKT, phospho-GSK3, phospho-ERK1/2, phospho-S6, c-Jun, Smurf1 and Smad1 were from Cell Signaling Technology (Beverly, MA, USA). Antibodies against ATF3, Sprr1a and Gadd45a were from Santa Cruz Biotechnology. All fluorescence-tagged secondary antibodies were from Molecular Probes, Inc. (Eugene, OR, USA). The siRNAs against Smad1 and Smurf1 (ON-TARGETplus SMART POOL) were from Thermo Scientific Dharmacon (Chicago, IL, USA). pCS2–hSmad1–EVE was from Addgene (plasmid 22993) [38] . The pCMV–EGFP–N1 plasmid was from Clontech, Inc. The dominant-negative PI3K construct was a mutant 85 kDa subunit of PI3K lacking the binding site for the catalytic 110 kDa subunit [49] , [54] . Animals All experiments involving animals were performed in accordance with the animal protocol approved by the Institutional Animal Care and Use Committee of the Johns Hopkins University. Eight to 10-week-old female CF-1 mice (weighing from 30 to 35 g) were purchased from Charles River Laboratories and housed in the University Animal Facility. The bax −/− mice were obtained from David Ginty (Johns Hopkins University). Primary culture of mouse adult DRG neurons DRGs from adult mice were dissected out and digested with collagenase A (1 mg ml −1 ) for 90 min, followed by trypsin-EDTA (0.05%) for 20 min at 37 °C. Enzyme-digested DRGs were washed three times with culture medium (MEM with L -glutamine, penicillin/streptomycin and 5% fetal calf serum) and dissociated with a 1 ml pipette tip in culture medium. The dissociated neurons were then centrifuged to remove the supernatant and plated into 24- or 12-well plates coated with a mixture of 100 μg ml −1 poly- D -lysine and 10 μg ml −1 laminin and was grown in culture medium described above without the addition of NGF or any other growth factors. After 3 days of culture, neurons were resuspended and replated on glass coverslips coated with a mixture of 100 μg ml −1 poly- D -lysine and 10 μg ml −1 laminin for overnight culture. Treatments denoted as ‘before replating’ indicate procedures in which neurons were first grown in the presence of a drug(s) of interest during the initial 3-day-culture period, but then the drug(s) was washed out at the time of replating. After washout and replating, neurons were grown in the absence of drug(s). Treatments denoted as ‘after replating’ indicate procedures in which neurons were first grown in the absence of a drug(s) of interest during the initial 3-day-culture period, but they were exposed to the drug(s) at the time of replating, followed by an overnight culture in the presence of the drug(s). For in vitro electroporation experiments, dissociated DRG neurons were centrifuged to remove the supernatant and resuspended in 80 μl of Amaxa electroporation buffer (for mouse neuron) with mixtures of siRNAs (0.2 nmol per transfection) and/or the EGFP (5 μg per transfection) plasmid. The suspended cells were then transferred to a 2.0-mm cuvette, followed by electroporation with the Amaxa Nucleofector apparatus. After electroporation, cells were immediately transferred to the desired volume of prewarmed culture medium and plated on culture dishes coated with a mixture of 100 μg ml −1 poly- D -lysine and 10 μg ml −1 laminin. After neurons fully attached to the substrates (4 h), medium was changed to remove the remnant electroporation buffer. After 3 days of culture, the cells were then resuspended and replated on glass coverslips with a mixture of 100 μg ml −1 poly- D -lysine and 10 μg ml −1 laminin. Replated adult DRG neurons were fixed with 4% paraformaldehyde (PFA) after overnight culture and then were subjected to immunocytochemistry. Measurement of axon growth All image analyses were performed with AxioVision 4.6 software (Carl Zeiss MicroImaging, Inc.) using the ‘measure/curve’ application. For quantification of axon length, neurons with processes longer than twice the diameter of cell bodies were photographed and the longest axon of each neuron was traced manually. In each experiment, ~100 neurons per condition were measured unless stated otherwise to calculate the mean value. At least three independent experiments were performed to compute the mean axon length and s.e.m. values, which were used to plot the bar graphs. Thus, ‘ n ’ in the bar graph indicates the number of independent experiments performed. For the in vivo axon regeneration experiments, the ‘ n ’ in the bar graph indicates the number of mice. To construct the cumulative distribution plots for the in vivo experiments, the lengths of all identifiable regenerating axons were pooled from multiple experiments. Thus, ‘ n ’ in the cumulative distribution plots indicates the number of total neurons analysed. Number of independent experiments performed and number of neurons analysed in each condition are depicted in the figures or in the legends. Quantitative real-time PCR For quantitative real-time PCR (qRT–PCR), total RNA was isolated with the TRI Reagent (Molecular Research Center) and RNA was reverse-transcribed by using Moloney murine leukaemia virus reverse transcriptase (Roche Applied Science). CFX96 real-time PCR detection system (Bio-Rad) was used for the quantification. The sequences of the forward and reverse primers were as follows: pten , 5′-TGGATTCGACTTAGACTTGACCT-3′ and 5′-TGGCGGTGTCATAATGTCTCT-3′; inpp4b 5′-TCAGGCGCTTGCTGGATTGGT and 5′-TGCCGACTGCCATGTCCTCCA; inpp5j 5′-CAAGTTCGCCATAGACAGCA and 5′-TTGTTGGTACCCACGTCAAA; smad1 , 5′-GACCGTGTATGAACTCACCAA-3′ and 5′-ATGCAGATGGATCTCAATCCA-3′; gap43 , 5′-AAGCAGCCAAGCTGAGGAG-3′ and 5′-AGTTCAGGCATGTTCTTGGT-3′. Compartmented cultures using two-compartment chambers The two compartmental chambers were provided by Dr. In Hong Yang [30] , [35] . The chambers were uniformly coated with a mixture of 100 μg ml −1 poly- D -lysine and 10 μg ml −1 laminin and DRG neurons were loaded into the somal compartment. Drugs were introduced into either the somal or the axonal side, as indicated, very slowly and carefully using a micropipette. Medium in the somal and axonal compartment was changed daily to re-establish the hydrostatic pressure difference between the somal and the axonal chambers to produce a fluid flow that prevents diffusion of drugs into the microchannels. Neurons cultured in different chambers were stained at the same time to quantify axons growing into the axonal compartment. In vivo electroporation of DRGs and sciatic nerve crush A 3-cm-long skin incision was made aseptically at the midline of the lower back after mice were anaesthetized. L4 or L5 were exposed, followed by injection of plasmid or siRNAs. Solution of plasmids (1.0 μl) or siRNAs were gradually injected into the DRG using a Picospritzer II (Parker Ins. ; pressure, 30 psi; duration: 8 ms) and electroporation was performed immediately after the injection using a custom-made tweezer-like electrode (Ø 1.2 mm) and a BTX ECM830 Electro Square Porator (five 15 ms pulses at 35 V with 950 ms interval). The wound was then closed and the mouse was allowed to recover. For nerve regeneration experiments, the sciatic nerve was exposed at the sciatic notch by a small incision 2 days after the in vivo electroporation. The nerve was then crushed and the crush site was marked with a size 10-0 nylon epineural suture. After surgeries, the wound was closed and the mice were allowed to recover. Three days after the sciatic nerve crush, the mice were terminally anaesthetized and transcardially perfused with PBS (pH 7.4), then with ice-cold 4% PFA in PBS. The whole sciatic nerves from the perfused animals were dissected out and postfixed overnight in 4% PFA at 4 °C. Before whole-mount flattening, it was confirmed that the place of epineural suture matched the injury site, and experiments were included in the analysis only when the crush site was clearly identifiable. Using whole-mounted tissue, all identifiable EGFP-labeled axons in the sciatic nerve were manually traced from the crush site to the distal growth cone to measure the length of axon regeneration. Immunohistochemistry and fluorescence imaging DRG tissues or dissociated neurons were lysed with RIPA buffer for 30 min on ice, followed by centrifugation at 10,000 g for 10 min at 4 °C. Proteins were separated on 4–12% gradient gels and transformed onto polyvinylidene fluoride (PVDF) membranes. After blocking with 5% non-fat milk, membranes were sequentially incubated with primary (overnight, 4 °C) and secondary antibodies (1–2 h, room temperature). Band intensity was quantified from three independent experiments using Image J software. Statistics Data are presented as mean±s.e.m. Two-tailed Student’s t -test was used to determine the statistical significance between different experimental groups, which was set at a value of P <0.05. How to cite this article: Saijilafu. et al. PI3K–GSK3 signalling regulates mammalian axon regeneration by inducing the expression of Smad1. Nat. Commun. 4:2690 doi: 10.1038/ncomms3690 (2013).